Characterization of the LCROSS impact plume from a ground-based imaging detection The Lunar CRater Observation and Sensing Satellite (LCROSS) mission was designed to search for evidence of water in a permanently shadowed region near the lunar south pole. An instrumented Shepherding Spacecraft followed a kinetic impactor and provided – from a nadir perspective – the only images of the debris plume. With independent observations of the visible debris plume from a more oblique view, the angles and velocities of the ejecta from this unique cratering experiment are better constrained. Here we report the first visible observations of the LCROSS ejecta plume from Earth, thereby ascertaining the morphology of the plume to contain a minimum of two separate components, placing limits on ejecta velocities at multiple angles, and permitting an independent estimate of the illuminated ejecta mass. Our mass estimate implies that the lunar volatile inventory in the Cabeus permanently shadowed region includes a water concentration of 6.3±1.6% by mass. The Lunar CRater Observation and Sensing Satellite (LCROSS) mission was designed to search for evidence of water in a permanently shadowed region near the lunar south pole [1] , [2] . The second stage of the rocket that launched LCROSS and the Lunar Reconnaissance Orbiter (LRO) was impacted into Cabeus crater on 09 October 2009 at 11:31:19.5 UTC to launch material (termed ‘ejecta’) from the subsurface and loft it into sunlight. An instrumented Shepherding Spacecraft (SSc) followed the impactor to obtain images and spectra of the debris plume from a nadir perspective before itself impacting into the Moon ~4 min later [3] , [4] . Although measurements from the SSc and LRO did successfully detect water lofted from the LCROSS impact [2] , [3] , [4] , [5] , [6] , the SSc provided the only visible images of the debris plume. Without an independent observation of the visible debris plume from a more oblique view, models of the morphology and dynamics of the ejecta from this unique cratering experiment are poorly constrained. The ultimate selection of Cabeus as the impact location was driven by the preponderance of hydrogen there – assumed to be associated with deposits of water ice – as measured by neutron spectrometers onboard the Lunar Prospector spacecraft [7] , [8] and LRO. The impact location was not ideal from an Earth-based perspective because a foreground hill obscured the impact site. This obscuration thus required material to ballistically rise above a height of 1.8 km in order to have been seen from Earth, thereby setting a strong limit on visible mass. Despite this limitation, a significant ground-based observing campaign was executed from the western United States and Hawaii to further characterize the LCROSS debris plume both spectroscopically and through imaging [9] . Aside from an enhancement of sodium in the lunar exosphere after the impact [10] , no other positive ground-based detections of the LCROSS debris plume were reported. Two groups reported non-detections from ground-based observations [11] , [12] . Here we report the first visible observations of the LCROSS ejecta plume from Earth, and thereby ascertain the morphology of the plume to contain a minimum of two separate components, place limits on ejecta velocities at multiple angles, and permit an independent estimate of the illuminated ejecta mass. Our mass estimate implies that the lunar volatile inventory in the Cabeus permanently shadowed region includes a water concentration of 6.3±1.6% by mass. Detection of the plume using principal component analysis In our initial paper [11] , we reported detection limits for the debris plume using Agile [13] on the Astrophysical Research Consortium (ARC) 3.5-m telescope at the Apache Point Observatory (APO) and a V-band filter coupled with a neutral density filter ( Fig. 1a ). We found that its V-band surface brightness had to be fainter than 9.5 magnitudes arcsecond −2 (mag arcsec −2 ) at 4 km above the impact point. Here, we present a unique analysis of these data using a new analytical approach. In order to search for a plume signal below the 3- σ detection limit set in ref. 11 , we employed a principal component analysis (PCA). PCA is a matrix factorization technique that finds statistically independent principal components (PCs) within a data set [14] . We applied PCA to our spatially and temporally resolved data (a time series), which yielded 961 PCs. We were able to identify the sources of the signals that are present in PCs 1–4 (see Methods). PCs 1 and 2 contained the static lunar landscape varying in dynamic range and in the size of the point spread function (PSF) due to atmospheric seeing. PCs 3 and 4 contained sub-pixel imperfections in image registration in orthogonal directions. PCs 1–4 were unwanted sources in the time series and were all statistically independent from any signal coming from the LCROSS plume. 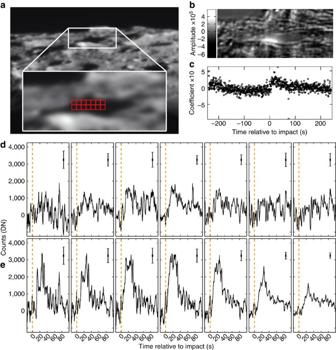Figure 1: Overview of the ground-based imaging detection of the LCROSS impact plume. (a) V-band image of Cabeus crater (flipped) at the south pole of the Moon as imaged with the Agile camera on the 3.5-m telescope at the APO in Sunspot, New Mexico, on the night of the LCROSS impact11. The inset shows the region used in our analysis with a red array overlaid to show the locations of 4 × 4-pixel photometry boxes used for the analysis of the detected plume signal. (b–c) PC20 of the observational data containing an unambiguous detection of the LCROSS impact plume. (b) The PC20 amplitudes show most of the visible debris (bright region). (c) The PC20 eigenvector is the time-varying strength of PC20. All data points in the eigenvector are represented by open diamonds and appear to be solid black where the diamonds overlap. All subsequent data shown includes PCs 5-961 unless otherwise noted. (d–e) Signal of the observed LCROSS plume for the photometry box array shown in (a). The vertical dashed lines in each photometry box denote the time of impact. Row (e) of photometry boxes is centred at 3.6 km above the impact site, and row (d) is at a height of 5.4 km. The vertical extent of the black bars in the upper right of each photometry box indicate the 1-σstandard deviation measured over a time range of −150 to −0.5 s relative to impact. Their horizontal extent represents the 2.5-s boxcar average applied to the data. Figure 1: Overview of the ground-based imaging detection of the LCROSS impact plume. ( a ) V-band image of Cabeus crater (flipped) at the south pole of the Moon as imaged with the Agile camera on the 3.5-m telescope at the APO in Sunspot, New Mexico, on the night of the LCROSS impact [11] . The inset shows the region used in our analysis with a red array overlaid to show the locations of 4 × 4-pixel photometry boxes used for the analysis of the detected plume signal. ( b – c ) PC20 of the observational data containing an unambiguous detection of the LCROSS impact plume. ( b ) The PC20 amplitudes show most of the visible debris (bright region). ( c ) The PC20 eigenvector is the time-varying strength of PC20. All data points in the eigenvector are represented by open diamonds and appear to be solid black where the diamonds overlap. All subsequent data shown includes PCs 5-961 unless otherwise noted. ( d – e ) Signal of the observed LCROSS plume for the photometry box array shown in ( a ). The vertical dashed lines in each photometry box denote the time of impact. Row ( e ) of photometry boxes is centred at 3.6 km above the impact site, and row ( d ) is at a height of 5.4 km. The vertical extent of the black bars in the upper right of each photometry box indicate the 1- σ standard deviation measured over a time range of −150 to −0.5 s relative to impact. Their horizontal extent represents the 2.5-s boxcar average applied to the data. Full size image Our PC20 ( Fig. 1b,c ) contained a clear signal from the LCROSS plume. However, owing to the nature of PCA, only portions of the plume with strong covariance in both space ( Fig. 1b ) and time ( Fig. 1c ) are described by any single PC. To extract the full spatial and temporal evolution of the plume’s signal in our data, we removed PCs 1–4, which were unambiguously unrelated to the plume, from the original time series. We refer to this removal of unwanted, known sources as PCA filtering (see Methods). We generated an array of brightness curves from our PCA-filtered data for pixels in the shadowed portion of Cabeus crater ( Fig. 1d,e ). These showed an unambiguous signal above the noise threshold (see Methods), with the strongest signal detected at the centre of the array ( Fig. 1e ) above the LCROSS impact site. Modelling the observed plume with synthetic plumes We explored the parameter space of possible plume morphologies and dynamics by comparing the array of brightness curves of the observed plume to those derived from a three-dimensional n -body ballistic plume model. Most early predictions for the LCROSS mission that were based on computational models and crater scaling relations [15] included a single plume component [16] , [17] . However, impact experiments conducted at the NASA Ames Vertical Range Gun in support of the LCROSS mission that used hollow projectiles demonstrated a bimodal ejecta plume structure consistent with the LCROSS SSc observations [4] , [18] . In these laboratory experiments, solid projectiles produced the standard, single-component plume (dubbed the ‘low-angle’ plume), whereas hollow projectiles produced a two-component plume (a ‘low-angle’ plus a ‘high-angle’ plume), with the low-angle plume excavating material from greater depths than the high-angle plume [18] . We tested both single- and multiple-component plume morphologies based on these results (which may be a parameterization of a continuum physical process). 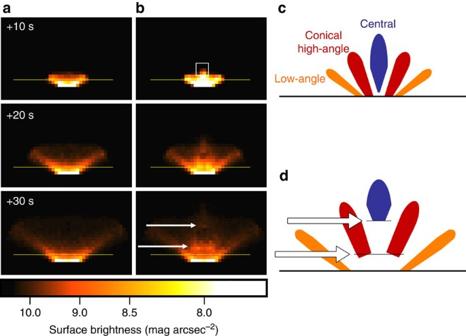Figure 2: Morphology of the synthetic plumes used to model the LCROSS impact plume. (a,b) Snapshots of two synthetic plumes at 10, 20, and 30 s after impact and (c,d) diagrams of the evolving plume morphology. (a) Images from our plume simulations with solely a low-angle plume component. Only illuminated particles that are above the local Sun height of 833 m at the LCROSS impact site are displayed. The yellow horizontal line indicates the height of the intervening foreground hill as seen from Earth. (b) Results from our best-match synthetic plume, which is comprised of both a low-angle plume and two-part high-angle plume. The arrows indicate the height of the slowest particles of the vertical part of the high-angle plume (top arrow) and the slowest particles of the conical part of the high-angle plume (bottom arrow). The white box in the uppermost image corresponds to the size (1.84 km on each side) and position of the bottom, centre photometry box (Fig. 1a, red array). (c) Illustrates a vertical cross-section ‘slice’ of the low-angle, conical high-angle, and central high-angle plume components. (d) Illustrates the lowest velocity particles in the conical and central high-angle plumes rising into our detection photometry boxes by 30 s after impact. Figure 2 shows sample synthetic plumes with and without a high-angle plume component. Figure 2: Morphology of the synthetic plumes used to model the LCROSS impact plume. ( a , b ) Snapshots of two synthetic plumes at 10, 20, and 30 s after impact and ( c , d ) diagrams of the evolving plume morphology. ( a ) Images from our plume simulations with solely a low-angle plume component. Only illuminated particles that are above the local Sun height of 833 m at the LCROSS impact site are displayed. The yellow horizontal line indicates the height of the intervening foreground hill as seen from Earth. ( b ) Results from our best-match synthetic plume, which is comprised of both a low-angle plume and two-part high-angle plume. The arrows indicate the height of the slowest particles of the vertical part of the high-angle plume (top arrow) and the slowest particles of the conical part of the high-angle plume (bottom arrow). The white box in the uppermost image corresponds to the size (1.84 km on each side) and position of the bottom, centre photometry box ( Fig. 1a , red array). ( c ) Illustrates a vertical cross-section ‘slice’ of the low-angle, conical high-angle, and central high-angle plume components. ( d ) Illustrates the lowest velocity particles in the conical and central high-angle plumes rising into our detection photometry boxes by 30 s after impact. Full size image We found that a synthetic plume consisting of a low-angle plume with ejection angles <45° with respect to the lunar surface, and an independent high-angle plume with ejection angles ranging from 50°–90° produced the best match to the observed brightness curves of Fig. 1d,e . No single-component synthetic plume could produce a match to all brightness curves in the array. This was consistent with the expectation that the LCROSS plume should be morphologically similar to those produced by hollow impactors. 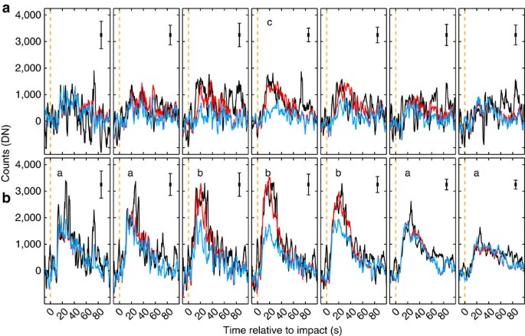Figure 3: Brightness curves of the observed LCROSS impact plume and synthetic plumes. Total 4 × 4 binned pixel counts of the observed LCROSS plume (black) and synthetic plumes (blue and red) as a function of time after impact for the photometry box array shown inFig. 1a. Row (b) of photometry boxes is centred at 3.6 km above the impact site, and row (a) is at a height of 5.4 km. The vertical extent of the black bars in the upper right of each photometry box indicate the 1-σstandard deviation for this box measured over two minutes of images prior to impact. Their horizontal extent represents the 2.5-s boxcar average applied to the observations and synthetic data. The blue lines are brightness curves for solely a low-angle plume component, corresponding to the plume shown inFig. 2a. We used the photometry boxes labelled ‘a’ to fit the parameters of the low-angle plume. The red lines are brightness curves for the best-match combined low and high-angle synthetic plume shown inFig. 2b. We used the boxes labelled ‘b’ to fit the parameters of the conical high-angle plume and the box labelled ‘c’ to fit the parameters of the central high-angle plume. Figure 3 shows an overlay of our observed LCROSS plume brightness curves (black) with results from two synthetic plumes – the best-match low-angle synthetic plume (blue), and the best-match synthetic plume with both low-angle and high-angle components (red). A single-component low-angle plume provides a match to the brightness curves in the photometry boxes labelled ‘a’ in Fig. 3 . This plume configuration produces a conical ‘inverted lampshade’ shape that expands with time as shown at 10, 20, and 30 s after impact in Figs 2a and 4c . Figure 3: Brightness curves of the observed LCROSS impact plume and synthetic plumes. Total 4 × 4 binned pixel counts of the observed LCROSS plume (black) and synthetic plumes (blue and red) as a function of time after impact for the photometry box array shown in Fig. 1a . Row ( b ) of photometry boxes is centred at 3.6 km above the impact site, and row ( a ) is at a height of 5.4 km. The vertical extent of the black bars in the upper right of each photometry box indicate the 1- σ standard deviation for this box measured over two minutes of images prior to impact. Their horizontal extent represents the 2.5-s boxcar average applied to the observations and synthetic data. The blue lines are brightness curves for solely a low-angle plume component, corresponding to the plume shown in Fig. 2a . We used the photometry boxes labelled ‘a’ to fit the parameters of the low-angle plume. The red lines are brightness curves for the best-match combined low and high-angle synthetic plume shown in Fig. 2b . We used the boxes labelled ‘b’ to fit the parameters of the conical high-angle plume and the box labelled ‘c’ to fit the parameters of the central high-angle plume. 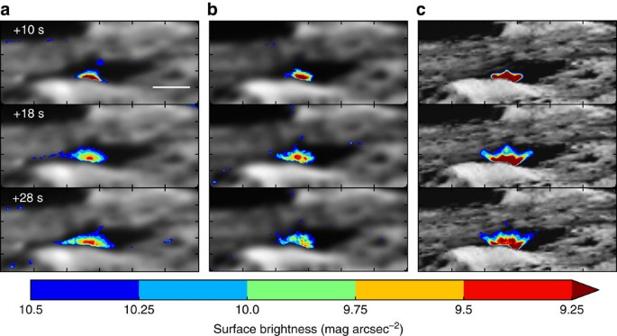Figure 4: Surface brightness contour maps of the observed plume and synthetic plume. Surface brightness contour maps of the LCROSS plume and a synthetic plume at 10, 18 and 28 s after impact. (a) Snapshots of the surface brightness for the plume signal extracted via PCA filtering from our observational data set superimposed over its PC1 amplitudes. The white scale bar represents a length of 10 km (21.74 pixels). (b) A simulated plume signal extracted via PCA filtering from the best-match synthetic data set superimposed over its PC1 amplitudes. (c) The best-match synthetic plume model as seen from above Earth’s atmosphere superimposed over the base lunar image. All columns have been smoothed with a 2.5-s boxcar average. SeeSupplementary Movie 1for data from all columns from times −10.0 to +59.5 s relative to impact. Full size image Figure 4: Surface brightness contour maps of the observed plume and synthetic plume. Surface brightness contour maps of the LCROSS plume and a synthetic plume at 10, 18 and 28 s after impact. ( a ) Snapshots of the surface brightness for the plume signal extracted via PCA filtering from our observational data set superimposed over its PC1 amplitudes. The white scale bar represents a length of 10 km (21.74 pixels). ( b ) A simulated plume signal extracted via PCA filtering from the best-match synthetic data set superimposed over its PC1 amplitudes. ( c ) The best-match synthetic plume model as seen from above Earth’s atmosphere superimposed over the base lunar image. All columns have been smoothed with a 2.5-s boxcar average. See Supplementary Movie 1 for data from all columns from times −10.0 to +59.5 s relative to impact. Full size image We note that the inverted lampshade shape of the model as seen from above the Earth’s atmosphere ( Fig. 4c ) does not match the PCA-extracted LCROSS plume shown in Fig. 4a . However, we found that atmospheric seeing distortions, which we replicated in our synthetic plume extraction procedure, smoothed the apparent shape of the synthetic plume extracted with our PCA filter ( Fig. 4b ). By increasing the standard deviation for low-angle particle ejection angles in our simulations to 10°, we could create a ‘fuzzier’ synthetic plume model morphologically similar to the shape in Fig. 4a (that is, so that Fig. 4c itself would look much like Fig. 4a ). However, owing to seeing-induced loss of resolution, synthetic plumes with differing low-angle standard deviation looked essentially identical after PCA extraction. In addition, we did not observe a noticeable difference in the extracted brightness curves for synthetic plumes with ejection angle standard deviation values from 3°–10° and therefore cannot constrain this parameter. We found that the time of peak brightness for the synthetic curves in Fig. 3 grid boxes labelled ‘a’ was sensitive to the average particle ejection angles, with the best-match angle to be 35±5° from horizontal, compared with the ~45° found experimentally for hollow projectiles fired into particulate targets [18] . These lower ejection angles are consistent with impacts into lower density, ‘fluffy’ target materials [18] . Our best-match low-angle plume ejection velocities ranged up to 500 m s −1 , although our results proved relatively insensitive to the upper limit. We could find no single-component synthetic plume that matched the LCROSS plume brightness curves in Fig. 3 grid boxes labelled ‘a’, ‘b’, and ‘c’ simultaneously. Matching the peak values for boxes ‘b’ and ‘c’ required the addition of separate high-angle plume components with different initial particle ejection angles and velocities from that of the low-angle plume. The red curves in Fig. 3 show results for the best-match combination of a low-angle plume and a high-angle plume, corresponding to the images in Fig. 2b . Our best-match synthetic plume morphology is illustrated in Fig. 2c,d . We found that a two-part high-angle plume was required to match our observed brightness curves for all the photometry boxes labelled ‘b’ and ‘c’ in Fig. 3 . This two-part plume consisted of a conical and central high-angle plume with separate ejection angles and initial particle velocities. Our best-match conical high-angle plume had random ejection angles between 55° and 75° and a particle velocity range of 150–400 m s −1 . This conical plume plus the low-angle plume provided a match to all observed plume photometry boxes labelled ‘a’ and ‘b’. Matching the curve in photometry box ‘c’ required an additional independent central high-angle plume with ejection angles from 75°–90° (that is, vertical) and particle velocities between 300 and 500 m s −1 . Results of laboratory impacts show that ejecta velocity drops off with increasing time after impact [18] . As a result, slower particles in the high-angle plume are inferred to originate at greater depths than those of the faster particles. The low velocity cutoffs for the conical and central high-angle plumes ( Fig. 2d ) may therefore represent either a drop off of ejected mass at lower velocities or possibly a sharp reduction in albedo for particles ejected at lower velocities and hence greater depths. We estimate that the particle albedo would have to drop by 75% at the lower ejection velocities to match our observed brightness curves. As this would imply an albedo as high as 0.3–0.6 for the shallower particles, we favour the possibility of a mass drop off below these lower velocity limits. We calculated the V-band surface brightness for the observed plume based on photometric calibrations outlined in ref. 11 (see Methods). We found the maximum plume brightness to be 10.0±0.1 mag arcsec −2 from 17–27 s after impact at a height of ~3.6 km above the impact point. This represents a lower brightness estimate for the LCROSS plume measured after losses due to atmospheric seeing and PCA filtering. We also converted the per-pixel brightness, or digital number (DN), values from our best-match simulation to surface brightness to estimate the maximum brightness of the LCROSS plume as seen from an Earth-based vantage point above the atmosphere. We calculated an initial peak in brightness owing to the rise of the central high-angle plume of 9.6±0.1 mag arcsec −2 from 11–13 s after impact. Our verification procedure showed that atmospheric seeing attenuated this narrow brightness peak (see Methods). The simulated plume displayed a second, broader brightness peak of 9.9±0.1 mag arcsec −2 from 18–28 s after impact. The size and shape of the observed and best-match synthetic plume at 10, 18, and 28 s is illustrated in Fig. 4 . Our detection proved possible only against the background of Cabeus crater as the signal-to-noise ratio (SNR) dropped off significantly outside of this dark region. The surface brightness in the floor of Cabeus crater was 6.75 mag arcsec −2 in V-band at the time of impact [11] . Any future attempt to image a similar event would require a plume background at or below this surface brightness value. We have therefore demonstrated the ability to detect and characterize a resolved ejecta plume 3.25 mag arcsec −2 fainter than the background using this PCA filtering technique. This result suggests limits for the maximum background brightness compatible with Earth-based imaging of any future lunar impact experiments. We determined the peak optical depth of the LCROSS plume based on the brightness of the synthetic plume before atmospheric losses between 18–28 s after impact (see Methods). We converted our plume simulation DN values to total particle cross-sectional area using a photometric transfer function [19] . We derived optical depth and mass estimates assuming a V-band lunar regolith albedo of 0.17 derived for highland material from lunar reflectance spectra [20] . Using this albedo, we estimated the peak optical depth with 1- σ uncertainties (see Methods) at the centre of the plume at a height of 3.6 km above the impact site (the centre ‘b’ box in Fig. 3 ) to be 0.0018±0.0002. We calculated the mass of all illuminated particles in the LCROSS plume at 20 s after impact based on our best-match simulation. Our detection grid extended down to only 2.7 km above the impact site owing to the scattered light from the bright foreground hill. However, using results from the best-match simulated plume, we extrapolated the total plume mass down to the sunlit horizon height of 833 m. This allowed us to compare our mass estimate to that published based on SSc images taken from above the plume [3] . Adopting the same assumptions [3] for an average particle radius of 2.5 μm and a particle density of 3,000 kg m −3 , and assuming a regolith albedo of 0.17, we estimated the total illuminated plume mass to be 2,240±400 kg. This is ~30% lower than the mass of 3,150±790 kg calculated based on spectra taken with the ultraviolet/visible spectrometer on the SSc for times 0–23 s post-impact [3] . Of this total, the high-angle plume represented 18% of the illuminated mass at 20 s after impact. The concentrations of water ice by mass in the regolith at the LCROSS impact site derived from our measurements of the plume mass – and based on the reported measurement of water mass for times 0–23 s post-impact from LCROSS SSc data [3] – is 6.3±1.6%. Observational data preparation We processed the original data from the ARC 3.5-m Agile instrument using standard techniques to remove the CCD bias, dark current, and pixel-to-pixel sensitivity variations. Forty-five minutes of continuous data (Agile is a frame-transfer CCD) were collected bracketing the LCROSS impact. A subset of those data covering 240 s before and after the impact time is analysed in this work. The observations were registered to sub-pixel accuracy by cross-correlating images apodized to the Cabeus crater area. PCA filtering The observational time series analysed in this work contains a brightness curve for every spatial pixel. PCA finds a set of orthogonal eigenvector brightness curves, which are called PCs, and the amplitude of each PC that is necessary to reproduce each pixel’s original brightness curve in the data, V , by a linear superposition of all PCs. This is a factorization into PC eigenvectors, H , and PC amplitudes, W , which can be represented as follows: where V is an m × r matrix that contains m brightness curves (pixels) sampled at r times (frames), W is an m × r matrix of the PC amplitudes, H is an r × r matrix of the PC eigenvectors, i denotes an individual pixel, τ denotes an individual time (frame) and a denotes an individual PC. The PCs are chosen so that the first PC is the brightness curve that yields the smallest residuals when, for each pixel, this brightness curve is multiplied by an arbitrary amplitude (positive or negative, because they describe the residuals in the original brightness curve that are left after accounting for each lower order PC) and subtracted from that pixel’s brightness curve. The second PC describes the strongest covarying brightness curve present in the residuals, which will necessarily be orthogonal to the brightness curve of the first PC. Higher order PCs are found until the number of PCs equals r , at which point the PCs constitute a complete set of basis vectors for the data’s r -dimensional time space. Therefore, a PCA of our time series effectively finds the brightness curves (PC eigenvectors) that describe decreasing amounts of covariance in the data. PC amplitudes describe the extent to which each brightness curve is present in each pixel of the image. The original brightness curve at an individual pixel is the sum of the pixel’s PC amplitude multiplied by the PC eigenvector over all PCs. As expected, the source of variance described by PC1 is the lunar landscape ( Fig. 5a ). The fact that the PC1 eigenvector ( Fig. 5e ) is not constant with time is due to variations in the atmospheric seeing, which results in a different dynamic range of the lunar landscape between frames. A frame with a PSF with a larger full-width-at-half-maximum (FWHM) will have some photons from the bright foreground hill blended into the crater shadow, resulting in an artificially brighter shadow and dimmer hill. The source for PC2 ( Fig. 5b,f ) is the blurring or sharpening of each frame with respect to the lunar landscape image of PC1, with negative eigenvector coefficients denoting sharpening. PCs 3 and 4 originate from sub-pixel imperfections in image registration in orthogonal directions ( Fig. 5c,d and g,h ), which are rotated ~12° clockwise from the image’s X - and Y -axes. This rotation arose from our decision to register all frames relative to a single reference frame that was apodized with a Gaussian centred on the point of the bright foreground hill directly above the impact point, which has a slope of the same angle. Therefore, errors in registration were highly correlated in directions either along the slope of the hill or orthogonal to it. Errors in these different directions were statistically independent. 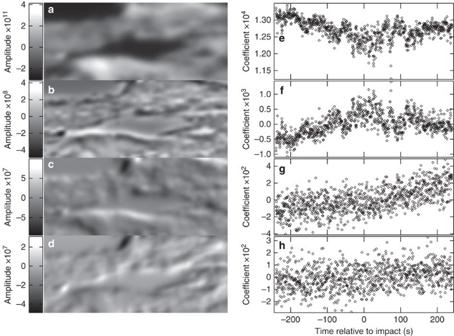Figure 5: Principal component analysis of the observations of the LCROSS impact. The four PCs containing unambiguous sources of variance in the observational data. All data points in the eigenvectors are represented by open diamonds and appear to be solid black where the diamonds overlap. (a) PC1 amplitudes show the most highly correlated image of the lunar landscape across all frames. (e) The PC1 eigenvector describes the variations in the dynamic range from frame to frame. (b) PC2 amplitudes show brightness variations from the largest-scale variations in atmospheric seeing. (f) The PC2 eigenvector describes the variations in the size of the PSF. (c) PC3 amplitudes show sub-pixel imperfections in image registration along a line approximately perpendicular to the foreground hill directly above the impact point. (g) The PC3 eigenvector describes the extent of the image offset in this direction. The PC4 amplitudes (d) and eigenvector (h) contain analogous information to PC3 but along a line approximately parallel to the same point on the foreground hill. Figure 5: Principal component analysis of the observations of the LCROSS impact. The four PCs containing unambiguous sources of variance in the observational data. All data points in the eigenvectors are represented by open diamonds and appear to be solid black where the diamonds overlap. ( a ) PC1 amplitudes show the most highly correlated image of the lunar landscape across all frames. ( e ) The PC1 eigenvector describes the variations in the dynamic range from frame to frame. ( b ) PC2 amplitudes show brightness variations from the largest-scale variations in atmospheric seeing. ( f ) The PC2 eigenvector describes the variations in the size of the PSF. ( c ) PC3 amplitudes show sub-pixel imperfections in image registration along a line approximately perpendicular to the foreground hill directly above the impact point. ( g ) The PC3 eigenvector describes the extent of the image offset in this direction. The PC4 amplitudes ( d ) and eigenvector ( h ) contain analogous information to PC3 but along a line approximately parallel to the same point on the foreground hill. Full size image Our thorough understanding of PCs 1–4 allowed us to remove these unwanted sources of correlated signal in order to make possible a low-SNR detection of the plume. We filtered out PCs 1–4 by reconstructing the original time series from its PCA factorization using only PCs 5–961. The contribution to the original data, X , from an arbitrary set of N PCs, A , can be found using where N≤r . The original time series can be perfectly reconstructed, without any loss of data, if A includes all PCs found in the PCA factorization. We created our filtered observational time series for plume detection, X filtered , using the set of PCs that may contain plume signal, A filtered =[5,6,…,961]. Thus, the extracted plume signal reported in this work contains the portion of the plume signal that is clearly present in PC20 ( Fig. 1b,c ) as well as any ambiguous or unrecognizable plume signal that is present in any of PCs 5–961. We subtracted an average image of pre- and post-impact frames (−240 to −0.5 s and +100 to +240 s relative to impact, respectively) from each frame of our PCA-filtered time series to account for any variations in the background counts of the static landscape after applying the PCA filter. To further increase the SNR, we applied a five-frame (2.5 s) boxcar average ( Supplementary Movie 1 , left panel). To produce the brightness curves seen in Fig. 1d,e , we binned our data spatially into a 2 × 7 array of 4 × 4-pixel photometry boxes ( Fig. 1a ), with each box being 1.04 arcsec (″) on a side, or 1.84 km at lunar distance considering Agile’s plate scale of 0.260″ per pixel. The array enclosed a region of 28 × 8 pixels; this corresponded to a region 7.28 × 2.08 km at the projected distance on the Moon. The bottom, centre photometry box was directly above the LCROSS impact point at the lowest altitude that was clear of the foreground hill from our viewing geometry. Validation of the plume detection method In order to determine if the detected signal in the PCA-filtered data came from the LCROSS ejecta plume, we developed a synthetic plume verification procedure to test the sensitivity of our PCA filtering method to artificial input brightness curves. PCs 1–4 were exceptionally similar between the real and synthetic data sets ( Figs 5 and 6 ), meaning that we successfully accounted for the sources of variance identified. 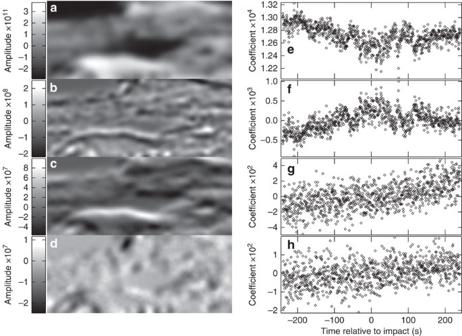Figure 6: Principal component analysis of synthetic observations of the synthetic plume. PCs 1–4 (a–h) of the best-match synthetic time series. Close agreement in the structure of these PCs and those of the observational data set (Fig. 5) shows that we correctly identify the dominant sources of variance in the data. The absolute range of each PC’s amplitudes is arbitrary and does not affect the resulting analysis. All data points in the eigenvectors are represented by open diamonds and appear to be solid black where the diamonds overlap. Figure 6: Principal component analysis of synthetic observations of the synthetic plume. PCs 1–4 ( a – h ) of the best-match synthetic time series. Close agreement in the structure of these PCs and those of the observational data set ( Fig. 5 ) shows that we correctly identify the dominant sources of variance in the data. The absolute range of each PC’s amplitudes is arbitrary and does not affect the resulting analysis. All data points in the eigenvectors are represented by open diamonds and appear to be solid black where the diamonds overlap. Full size image To assess the plume parameters, we first created an array of input brightness curves representing a possible plume ( Fig. 7 , green lines). We then created synthetic observations of this hypothetical pristine plume signal as described below. These synthetic observations were analysed using the same PCA filtering algorithm and binning used to produce the observed LCROSS plume brightness curves, and the brightness curves of the observations and simulations were then compared. The indigo lines in Fig. 7 show the synthetic brightness curves after addition of artificial atmospheric distortion only, which even a best-case detection of the synthetic plume signal would include. The red lines in Fig. 7 are the resulting plume signal extracted from the synthetic observations. Comparison to the plume signal extracted from the real observations ( Fig. 1d,e ) confirmed that our detection was in fact consistent with an ejecta plume. Details of the synthetic data creation process are presented in the following sections. 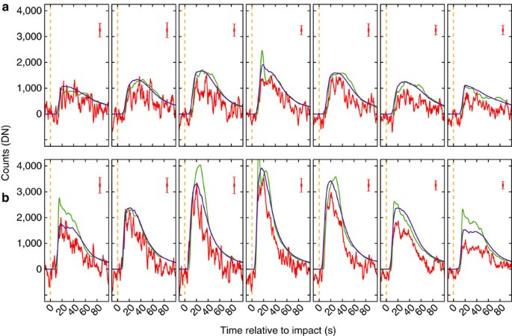Figure 7: Effects of Earth’s atmosphere and noise on a synthetic plume’s brightness curve. Total 4 × 4 binned pixel counts of a synthetic plume for the array of photometry boxes shown inFig. 1a. Row (b) of photometry boxes is centred at 3.6 km above the impact site, and row (a) is at a height of 5.4 km. The vertical dashed lines in each photometry box denote the time of impact. The green lines are the brightness curves of the light from the synthetic plume prior to entering Earth’s atmosphere. The indigo lines are the brightness curves of the synthetic plume after atmospheric seeing distorts the light. The red lines are the extracted brightness curves of the synthetic plume (using our PCA filtering method) from synthetic observations that contained the lunar landscape, synthetic plume, atmospheric seeing, and noise. The vertical extent of the red bars in the upper right of each photometry box indicate the 1-σstandard deviation for the extracted brightness curves (red lines) for this box measured over two minutes of synthetic images prior to impact. Their horizontal extent represents the 2.5-s boxcar average applied to the synthetic data. Figure 7: Effects of Earth’s atmosphere and noise on a synthetic plume’s brightness curve. Total 4 × 4 binned pixel counts of a synthetic plume for the array of photometry boxes shown in Fig. 1a . Row ( b ) of photometry boxes is centred at 3.6 km above the impact site, and row ( a ) is at a height of 5.4 km. The vertical dashed lines in each photometry box denote the time of impact. The green lines are the brightness curves of the light from the synthetic plume prior to entering Earth’s atmosphere. The indigo lines are the brightness curves of the synthetic plume after atmospheric seeing distorts the light. The red lines are the extracted brightness curves of the synthetic plume (using our PCA filtering method) from synthetic observations that contained the lunar landscape, synthetic plume, atmospheric seeing, and noise. The vertical extent of the red bars in the upper right of each photometry box indicate the 1- σ standard deviation for the extracted brightness curves (red lines) for this box measured over two minutes of synthetic images prior to impact. Their horizontal extent represents the 2.5-s boxcar average applied to the synthetic data. Full size image Creation of a base lunar image We began with a high quality digital rendering of the Moon with appropriate Earth viewing geometry at the time of impact, provided by Ernie Wright at NASA GSFC’s Scientific Visualization Studio. The rendering used Lunar Orbiter Laser Altimeter data and a lighting and shadow model to simulate the appearance of the Cabeus crater area up to an altitude of 200 km from the surface as viewed from the ARC 3.5-m telescope in Sunspot, New Mexico. We rotated the rendering (180° anticlockwise) to our preferred orientation of the scene, approximately matched the dynamic range of our observations, and then resized to match our observational plate scale (as measured by several oblique crater diameters). A final small rotation was applied (6.5° anticlockwise) to precisely match the observations. Creation of a synthetic data set A time series covering the same duration as the plume simulation was constructed using the image described in the previous section as a base. Frames from the plume simulation were added at the proper spatial and temporal locations, and a binary mask was then applied to each image to ensure that the obscuration from the foreground hill in the observations was replicated. To simulate the seeing experienced by Agile at the telescope, we scaled the PC2 eigenvector of the observational data set to a range of FWHMs appropriate to replicate the observational seeing. The range of FWHMs were chosen based on both visual inspection of the observations as well as information recorded by the Differential Image Motion Monitor (DIMM) at the APO. Unfortunately, DIMM measurements stopped shortly before the LCROSS impact due to the onset of twilight. Visual inspection of the synthetic and real observation images as well as comparisons between PC2 amplitudes ( Figs 5b and 6b ) matched well, with FWHMs ranging between 1.0 and 1.5″. A small amount of noise, ellipticity (up to 2%), and rotation were added to the PSFs before convolution with the synthetic data set to better simulate a realistic PSF. These additions have only a small discernible impact on the appearance of the plume signal as seen in our reconstructions but better match the fraction of total variance accounted for by each PC. Additional noise sources considered After this ‘roughed up’ PSF was convolved into the synthetic observation, a constant bias of 3,000 DN was added to simulate large-scale scattered light from the Moon. Although a more Gaussian distribution centred on the illuminated portion of the Moon that is visible from Earth is likely more applicable, our observations are on a small enough scale for this to be a small effect. Spot checks of the minimum brightness of dark craters in our observations revealed 3,000 DN to be roughly representative of the brightness floor, not falling sharply until the dark sky well outside the lunar limb and our sub-frame used in the analysis ( Fig. 1a ). Poisson and read noise from the Agile camera were added next, with care taken to add them both in terms of electrons (e − ) by dividing the image by the camera gain setting (1.93 DN per e − ). Random Poisson noise ( ) was added first, followed by adding Gaussian randomized read noise (6.62 e − ) before converting the observation back to DN by multiplying by the gain factor. At this point, the values in the synthetic observation image were truncated to an unsigned 16-bit range (0–65,535) to prevent integer overflows. As the image registration utilized apodization focused on the bright, high contrast, sloped foreground hill, image shifts derived from PCs 3 and 4 were relative to that slope. Sub-pixel shifts not accounted for during image alignment are visible as elongated and/or ‘embossed’ crater edges ( Fig. 5c,d ) in those PCs. To replicate this, we rotated our synthetic observations (12° anticlockwise) before applying sub-pixel shifts independently in the X (PC4) and Y (PC3) directions. We used rescaled versions of PCs 3–4 amplitudes (0–0.2 pixels) from the observational data set to shift our synthetic observations. Too large of a shift ( ) could lead (after interpolation) to a shift of an entire pixel, which was clearly not seen in our observations after alignment. The shifts were applied by means of a 2-D polynomial transform, after which we derotated the image to return to the orientation seen by Agile. After one final check to make sure that rotation/interpolation had not pushed any pixel values past the unsigned 16-bit limit, the synthetic observation was written to disk and the process was repeated until the synthetic time series was complete. On a server with AMD Opteron 6172 processors, this process wrote a synthetic observation to disk approximately every 0.5 s. This does not take into account the time to create the ballistic plume simulation, which completed in ~10 min on the same machine; neither operations were significantly multithreaded. Plume modelling Our plume model assigned initial velocities and ejection angles to ~200,000 particles at the time of impact and tracked their trajectories individually throughout the time of our observations. The low-angle plume particles were assigned ejection velocities and angles according to scaled values derived from laboratory experiments of impacts at similar velocities [18] . Our model allowed for adjusting the relative particle density of the low-angle and high-angle plumes as well as specifying separate mass–velocity and mass–angle relationships for the two components. From these simulations, we extracted brightness maps of the plume at 0.5 s intervals binned to a resolution of 0.46 km to match our Agile image frame rate and spatial resolution. We interpreted each simulated particle as a unit of brightness, or DN, and found through iterative simulation the number of total plume DN needed to match our observed brightness curves. The raw science and calibration images are archived in NASA’s Planetary Data System, Volume ID: lunar01/ear-l-apo35m_agile-2-edr-lcross-v1/lcragi_0xxx/. All codes relevant to PCA filtering and synthetic observation generation are being prepared for submission to NASA’s Planetary Data System. Derivation of optical depth and mass We based our calculation of optical depth and plume mass on the reflectivity relationship adapted from equation 5 (ref. 19 ): where is the reflectivity of the individual plume particles, a is the Sun–Moon distance at the time of the LCROSS impact, Δ is the Earth–Moon distance, A is the Sun–Earth distance, A reg is the total cross-sectional area of plume (regolith) particles per unit area, m reg is the V-band magnitude of the total regolith particles in the unit area, and m sun is the V-band magnitude of the Sun. From JPL Horizons, Δ=3.6712 × 10 5 km and a≈A . In V-band, m sun =−26.75 (ref. 21 ). The calibrated zero-point magnitude for the Agile images was given in equation of ref. 11 as: with counts, x , in DN per pixel and exposure time, t exp , in seconds. Setting t exp =0.5 and adopting this magnitude as the magnitude of plume particles in a unit area equal to a projected pixel at the Moon, m reg : Combining these relations yields the following expression for the total cross-sectional area of plume particles in a projected pixel in square metres: For low optical depth ( τ <<1), τ is approximately equal to the cross-sectional area of all particles in a pixel divided by the projected area of a pixel, A pix , at the Moon. The Agile plate scale is 0.260″ per pixel, which is 460 m at the Moon. Therefore, τ is given by We assumed a regolith particle for highland material based on lunar regolith reflectance spectra [20] . At the V-band central wavelength of 0.55 μm, this value is 0.17. Therefore, the expression for optical depth becomes: For our best-match simulation, the DN per pixel in the bottom, centre photometry box of Fig. 3 labelled ‘b’ at 24 s after impact was 239±25, which results in an optical depth of The total mass of all illuminated plume particles, M plume , is the product of the mass of a single plume particle, M part , and the total number of plume particles, η part : In these simulations, each simulated particle was counted as one DN and the total number of DN, DN plume , was set such that the peak intensity of synthetic plume brightness curves matched those of the observed plume. We divide equation (6) by x , to get the plume’s cross-sectional area per DN, A DN . The total number of plume particles equals: with cross-sectional area of a particle given by A part , and so The mass of a particle is given by M part =(4/3) πρ , where ρ is the particle density, assumed here to be 3,000 kg m −3 . A part = π , therefore and combining equations (12) and (13) yields: If we assume an average particle radius of 2.5 μm to compare to mass estimates from the LCROSS SSc [3] , we get the following: For a value of of 0.17 for highland regolith, the total illuminated mass becomes: For our best-match simulation, the total DN above 833 m at 20 s after impact was 140,000±26,000, which results in a total illuminated mass of Our calculated mass of 2,240±400 kg is ~30% lower than the estimated plume mass of 3,150±790 kg for times 0–23 s post-impact based on spectra taken from above the impact site with the ultraviolet/visible spectrometer on the LCROSS SSc [3] . This estimated mass derived from Equation (15) is linearly dependent on both the estimates for particle density, ρ , and particle radius, R part , and inversely proportional to the estimated ejecta albedo. Therefore, assuming a regolith consisting of irregular grains with an effective density of 2,000 kg m −3 , would result in a lower plume mass estimate of 1,500±270 kg. On the other hand, assuming a larger average particle radius or darker material on the floor of Cabeus crater would increase this mass estimate. We estimate the concentration of water ice by mass in the regolith at the LCROSS impact site by using our simulation results for 20 s after impact and the LCROSS SSc measurement of total water mass for times 0–23 s post-impact of M water =141±26 kg (ref. 3 ), yielding Our concentration estimate is ~40% higher than that derived from the LCROSS SSc data [3] for times 0–23 s post-impact of 4.5±1.4%. Their result for the times 0–23 s post-impact is a more appropriate value for comparison to our results at 20 s post-impact than their average result during times 0–180 s post-impact, which was 5.6±2.9%. How to cite this article: Strycker, P.D. et al . Characterization of the LCROSS impact plume from a ground-based imaging detection. Nat. Commun. 4:2620 doi: 10.1038/ncomms3620 (2013).